Atom–light interactions in photonic crystals The integration of nanophotonics and atomic physics has been a long-sought goal that would open new frontiers for optical physics, including novel quantum transport and many-body phenomena with photon-mediated atomic interactions. Reaching this goal requires surmounting diverse challenges in nanofabrication and atomic manipulation. Here we report the development of a novel integrated optical circuit with a photonic crystal capable of both localizing and interfacing atoms with guided photons. Optical bands of a photonic crystal waveguide are aligned with selected atomic transitions. From reflection spectra measured with average atom number , we infer that atoms are localized within the waveguide by optical dipole forces. The fraction of single-atom radiative decay into the waveguide is Γ 1D /Γ′ ≃ (0.32±0.08), where Γ 1D is the rate of emission into the guided mode and Γ′ is the decay rate into all other channels. Γ 1D /Γ′ is unprecedented in all current atom–photon interfaces. Localizing arrays of atoms in photonic crystal waveguides (PCW) with strong atom–photon interactions could provide new tools for quantum networks [1] , [2] , [3] and enable explorations of quantum many-body physics with engineered atom–photon interactions [4] , [5] , [6] , [7] , [8] , [9] , [10] , [11] , [12] , [13] , [14] , [15] , [16] , [17] , [18] , [19] . Bringing these scientific possibilities to fruition requires creation of an interdisciplinary ‘toolkit’ from atomic physics, quantum optics and nanophotonics for the control, manipulation and interaction of atoms and photons with a complexity and scalability not currently possible. Important initial advances to integrate atomic systems and photonics have been made within the setting of cavity quantum electrodynamics with atom–photon interactions enhanced in micro- and nanoscopic optical cavities [20] , [21] , [22] , [23] , [24] , [25] , [26] and waveguides [27] , [28] , [29] . At a minimum, the further migration to photonic crystal structures should allow the relevant parameters associated with these paradigms to be pushed to their limits [26] and greatly facilitate scaling. For example, modern lithographic processing can create nanoscopic dielectric waveguides and resonators with optical quality factors Q >10 6 and with efficient coupling among heterogeneous components [30] , [31] , [32] , [33] , [34] , [35] . A more intriguing possibility that has hardly been explored is the emergence of completely new paradigms beyond the cavity and waveguide models, which exploit the tremendous flexibility for modal and dispersion engineering of PCWs. For example, the ability to tune band edges near atomic transition frequencies can give rise to strongly enhanced optical interactions [36] , [37] , [38] , [39] , [40] . This enables a single atom to exhibit nearly perfect emission into the guided modes (Γ 1D ≫ Γ′) and to act as a highly reflective mirror (for example, reflection | r 1 | ≳ 0.95 and transmission | t 1 | ≲ 0.05 for one atom [41] ). The entanglement of photon transport with internal states of a single atom can form the basis for optical quantum information processing [1] , [2] , [3] with on-chip quantum optical circuits. At the many-body level, the strong interplay between the optical response and large optical forces of many atomic ‘mirrors’ can give rise to interesting optomechanical behaviour, such as self-organization [15] . Even more remarkable phenomena in PCWs arise when atomic frequencies can be tuned into photonic band gaps, including the ability to control the range, strength and functional form of optical interactions between atoms [4] , [16] , [17] , [18] . For example, atoms trapped near otherwise perfect photonic crystal structures can act as dielectric defects that seed atom-induced cavities [18] and thereby allow atomic excitations to be exchanged with proximal atoms [16] . The atom-induced cavities can be dynamically controlled with external lasers enabling the realization of nearly arbitrary long-range spin Hamiltonians and spatial interactions (such as an effective Coulomb potential mediated by PCW photons) [18] , providing a novel tool for quantum simulation with cold atoms. Control over PCW dispersion is also expected to facilitate novel atomic traps based upon quantum vacuum forces [19] , [41] , [42] . The prerequisite to all of these possibilities is a designable platform that allows the simultaneous alignment of optical bands for optical trapping and for interaction physics with atoms, which we demonstrate here for the first time. Here, we report advances that provide rudimentary capabilities for such a ‘toolkit’ with atoms coupled to a PCW. As illustrated in Fig. 1 , we have fabricated the integrated optical circuit with a photonic crystal whose optical bands are aligned with atomic transitions for both trapping and interfacing atoms with guided photons [41] , [43] . The quasi-1D PCW incorporates a novel design that has been fabricated in silicon nitride (SiN) [43] , [44] (Methods) and integrated into an apparatus for delivering cold caesium atoms into the near field of the SiN structure. From a series of measurements of reflection spectra with atoms coupling to the PCW, we infer that the rate of single-atom radiative decay into the waveguide mode is Γ 1D ≃ (0.32±0.08)Γ′, where Γ 1D is the emission rate without enhancement or inhibition due to an external cavity and Γ′ is the radiative decay rate into all other channels. The corresponding single-atom reflectivity is | r 1 | ≃ 0.24, representing an optical attenuation for one atom greater than 40% [12] , [41] . For comparison, atoms trapped near the surface of a fused silica nanofiber exhibit Γ 1D ≃ (0.04±0.01)Γ′ (refs 27 , 28 , 29 ), comparable with observations with atoms and molecules with strongly focused light [45] , [46] . By comparing with numerical simulations, our measurements suggest that atoms are guided to unit cells of the PCW by optical dipole forces. 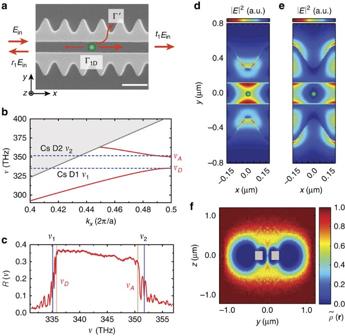Figure 1: Design and characterization of a 1D PCW. (a) SEM image of the APCW made from 200-nm thick (alongz-axis) SiN (ref.43). Arrows indicate radiative processes of an atom (green circle) coupled to an incident electric fieldEin. Scale bar, 500 nm. (b) Calculated band structure of fundamental TE-like modesE1,E2(red solid lines), with dominant electric field polarized in they-direction. The dashed lines mark the frequenciesν1andν2of the caesium D1, D2lines, respectively. (νA,νD) mark near the band edge. The gray solid line marks the light line. (c) Measured reflection spectrum with fast fringe removed (Methods) around the band gap shown in (b). (d) |E|2cross-sections ofE2mode nearν2, and (e)E1mode nearν1within a unit cell calculated with the MPB software package57(Methods). Both modes are polarized with their primary electric field component in the in-planey-direction. (f) Simulated relative densityof atoms in thex=0 plane of (e) with the optimal excitation of the blue-detunedE1mode atkx=π/a(see text). Figure 1: Design and characterization of a 1D PCW. ( a ) SEM image of the APCW made from 200-nm thick (along z -axis) SiN (ref. 43 ). Arrows indicate radiative processes of an atom (green circle) coupled to an incident electric field E in . Scale bar, 500 nm. ( b ) Calculated band structure of fundamental TE-like modes E 1 , E 2 (red solid lines), with dominant electric field polarized in the y -direction. The dashed lines mark the frequencies ν 1 and ν 2 of the caesium D 1 , D 2 lines, respectively. ( ν A , ν D ) mark near the band edge. The gray solid line marks the light line. ( c ) Measured reflection spectrum with fast fringe removed (Methods) around the band gap shown in ( b ). ( d ) | E | 2 cross-sections of E 2 mode near ν 2 , and ( e ) E 1 mode near ν 1 within a unit cell calculated with the MPB software package [57] (Methods). Both modes are polarized with their primary electric field component in the in-plane y -direction. ( f ) Simulated relative density of atoms in the x =0 plane of ( e ) with the optimal excitation of the blue-detuned E 1 mode at k x = π / a (see text). Full size image Design and characterization of a 1D photonic crystal waveguide Turning to our experiment, we begin with a scanning electron microscope (SEM) image of a small section of our 1D PCW shown in Fig. 1a . The device consists of two parallel nanobeams with sinusoidal modulation at the outer edges (an ‘alligator’ PCW or APCW). A challenge in the fabrication of PCWs for atomic physics is placement of the band edges near relevant atomic transition frequencies. Our APCW design facilitates this juxtaposition by fine tuning the gap between the parallel nanobeams and the amplitude of sinusoidal modulation in the APCW. Figure 1b shows the band structure of two fundamental transverse electric (TE-like) modes calculated based on the dimensions measured from SEM images as in Fig. 1a . The two blue dashed lines correspond to the transition frequencies of the Cs (D 1 , D 2 ) lines at ( ν 1 =335, ν 2 =351) THz ((895, 852) nm) that straddle the band edge frequencies ( ν D , ν A ) at k x = π / a for the lower (dielectric) and upper (air) TE bands, respectively. To validate these results, we measure the reflection spectrum R ( ν ) versus the input frequency ν for the actual device used in the reported experiments; see Fig. 1c . The large reflectivity ( R ~0.35) from ν D to ν A corresponds to the band gap for the APCW, while the vertical dashed lines mark ( ν 1 , ν 2 ) just outside the band gap. Absent propagation loss to and from the APCW, we infer R gap ≃ 0.99 from measurements and numerical simulation. Beyond band edge placement, another requirement for realizing strong atom–light interactions in PCWs is to localize atoms in a region of high mode intensity within a unit cell. The use of two bands enables the separate engineering of the modes for trapping (lower band) and control of spontaneous emission (upper band). The blue-detuned E 1 mode excited at ν 1 in Fig. 1e can guide atoms into the centre of the vacuum space near regions of large | E 2 | 2 , with then a field near ν 2 in Fig. 1d serving as a probe mode. The efficacy of this strategy is supported by trajectory calculations of free-space atoms surrounding the APCW (Methods). As shown in Fig. 1f , atoms are guided from free space into the region of high | E 2 | 2 , resulting in a density ~30% of the remote free-space density. For the simulations, the Casimir–Polder potential for the structure in Fig. 1a is computed numerically following ref. 41 . The optical dipole potential is calculated using a guided mode at k x = π / a with total power of 1 μW and 10 GHz blue-detuning from the F =4↔ F ′=4 transition frequency of the D 1 line. An overview of the integrated APCW device is presented in Fig. 2 , and shows the optical pathways for excitation to and from the APCW, as well as the supporting structures of the SiN device to a silicon substrate. The entire APCW contains 260 unit cells with a lattice constant a =371 nm, and is terminated on each end by a mode matching section of 40 cells with tapered sinusoidal modulation and a transition section from a double- to a single-nanobeam waveguide. Input to and output from the device is achieved through an optical fibre butt-coupled to one of the single-nanobeam waveguides [44] (Methods). The one-way efficiency for propagation from the APCW to the fibre mode is T wf ≃ 0.6. To integrate the device into a cold atom apparatus, the silicon chip in the inset of Fig. 2a and its coupling optical fibres are mounted on a vacuum feedthrough with linear translation and rotation stages and inserted into a UHV chamber. Caesium atoms are delivered to the region surrounding the APCW by a three-stage process of transport and cooling (Methods). The resulting atomic cloud has a peak number density of ρ 0 ≃ 2 × 10 10 cm −3 at temperature T ≃ 20 μK measured via time-of-flight absorption imaging. 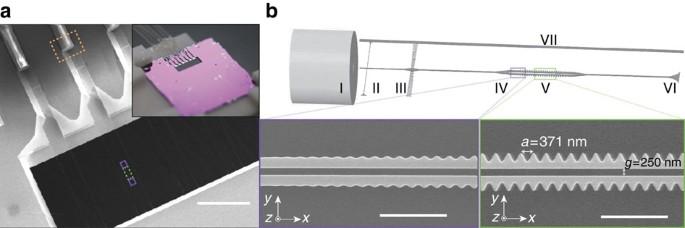Figure 2: Overview of the integrated APCW device. (a) SEM image of the silicon chip showing an integrated optical fiber (orange box) coupled, via a SiN nanobeam waveguide, to the APCW region (purple and green boxes). The APCW is located within a 1 × 3 mm through window (black region without dielectrics) where free-space atoms and cooling lasers are introduced. Inset shows a picture of the chip and the optical fibers glued to a vacuum-compatible holder. Scale bar, 0.5 mm. (b) Detailed schematic of the suspended SiN waveguide. Light enters the system via the optical fibre (I) butt-coupled44to the free end of the waveguide (II) which is supported by a tether array (III). Near the centre of the through window, the waveguide transitions into a double nanobeam, followed by tapering (IV) and APCW (V) sections, and again tapers out to terminate into the substrate (VI). Two parallel rails are added symmetrically to support the structure (one rail is illustrated in VII). The insets, corresponding to the purple and green boxes in (a), show SEM images of segments of the tapering (IV) and APCW (V) sections, respectively. Scale bars in IV and V, 2 μm. Figure 2: Overview of the integrated APCW device. ( a ) SEM image of the silicon chip showing an integrated optical fiber (orange box) coupled, via a SiN nanobeam waveguide, to the APCW region (purple and green boxes). The APCW is located within a 1 × 3 mm through window (black region without dielectrics) where free-space atoms and cooling lasers are introduced. Inset shows a picture of the chip and the optical fibers glued to a vacuum-compatible holder. Scale bar, 0.5 mm. ( b ) Detailed schematic of the suspended SiN waveguide. Light enters the system via the optical fibre (I) butt-coupled [44] to the free end of the waveguide (II) which is supported by a tether array (III). Near the centre of the through window, the waveguide transitions into a double nanobeam, followed by tapering (IV) and APCW (V) sections, and again tapers out to terminate into the substrate (VI). Two parallel rails are added symmetrically to support the structure (one rail is illustrated in VII). The insets, corresponding to the purple and green boxes in ( a ), show SEM images of segments of the tapering (IV) and APCW (V) sections, respectively. Scale bars in IV and V, 2 μm. Full size image Atom–light coupling in the APCW We study atom–light interactions in the APCW by first shutting off the cooling laser, followed by a delay of 0.1 ms and then interrogating the APCW with atoms by sending a guided probe pulse E probe of frequency ν p in the E 2 mode, with typical power ≃ 1 pW and measuring a reflected pulse of rE probe ; see Fig. 3a and Methods. Reflection spectra R (Δ p ) are recorded for 1 ms with a single-photon avalanche photodiode as a function of detuning Δ p = ν p − ν 2 a , where v 2 a is the free-space F =4↔ F ′=5 transition frequency of the D 2 line. For 10 ms following termination of the probe pulse, the atom cloud disperses, and then reference spectra R 0 (Δ p ) are recorded for a second probe pulse for 1 ms. For all experiments, the guided mode E 1 is driven continuously with power ≃ 0.6 μW at 10 GHz blue-detuning from the F =4↔ F ′=4 transition of the D 1 line. 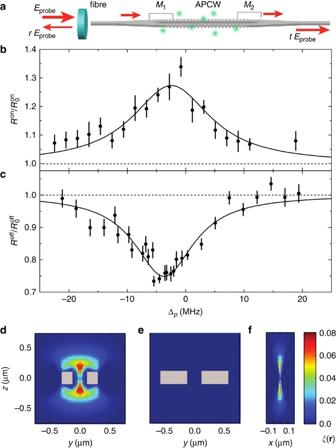Figure 3: Atom–light coupling in the PCW section. (a) Simplified schematic of a fiber-coupled PCW for reflection measurements with atoms (green dots). Dashed lines, marked asM1andM2, illustrate the mirrors for the effective low finessecavity formed by the tapered matching sections. (b,c) Measured reflection spectra (circles) with (b) an on-resonant cavity and (c) an off-resonant cavity in the APCW. Solid lines are Lorentzian fits with (b) linewidth of 15.2±1.8 MHz, peak reflectivitywhere the reflectivity with no atoms isand frequency shift Δ0=−2.5±0.6 MHz, and (c) linewidth of 11.5±1.1 MHz,where the reflectivity with no atoms isand Δ0=−3.7±0.3 MHz. Error bars for the data points reflect 1 s.d. estimated from the statistical uncertainties. (d) Simulatedin thex=0, (e)x=a/2, and (f)y=0 planes, with a guided potential ofmF=0 using the experimentally excited blue-detunedE1mode atkx=0.99π/a. Due to the deviation from the band edge, a small bump in the optical potential at the centre of the unit cells leads to atomic localization near the maxima ofin (d,f); see text and Methods for details. Masked areas in gray represent the APCW. Figure 3: Atom–light coupling in the PCW section. ( a ) Simplified schematic of a fiber-coupled PCW for reflection measurements with atoms (green dots). Dashed lines, marked as M 1 and M 2 , illustrate the mirrors for the effective low finesse cavity formed by the tapered matching sections. ( b , c ) Measured reflection spectra (circles) with ( b ) an on-resonant cavity and ( c ) an off-resonant cavity in the APCW. Solid lines are Lorentzian fits with ( b ) linewidth of 15.2±1.8 MHz, peak reflectivity where the reflectivity with no atoms is and frequency shift Δ 0 =−2.5±0.6 MHz, and ( c ) linewidth of 11.5±1.1 MHz, where the reflectivity with no atoms is and Δ 0 =−3.7±0.3 MHz. Error bars for the data points reflect 1 s.d. estimated from the statistical uncertainties. ( d ) Simulated in the x =0, ( e ) x = a /2, and ( f ) y =0 planes, with a guided potential of m F =0 using the experimentally excited blue-detuned E 1 mode at k x =0.99 π / a . Due to the deviation from the band edge, a small bump in the optical potential at the centre of the unit cells leads to atomic localization near the maxima of in ( d , f ); see text and Methods for details. Masked areas in gray represent the APCW. Full size image In the ideal case of a single atom in an infinite PCW, an incident probe beam would be reflected with amplitude coefficient | r 1 |=Γ 1D /(Γ 1D +Γ′), [12] where Γ 1D refers to emission into the guided mode of the APCW from the F =4↔ F ′=5 transition of the Cs D 2 line. Strong spontaneous decay into the guided mode (and hence large | r 1 |) results from the small area over which the guided mode is concentrated together with a reduced group velocity. These two effects are incorporated into an effective mode area for an atom at location within the APCW, namely , where n g ≃ 2 is the measured group index at ν 2 , σ =1.4 × 10 −9 cm 2 is the free-space atom–photon cross-section for an unpolarized atom, and Γ 0 is the free-space rate of decay. For unpolarized atoms located at the centre of a unit cell in the APCW, we expect A m ( 0 )=0.24 μm 2 , and hence | r 1 | ≃ 0.39, where Γ′ ≃ 0.9Γ 0 from numerical calculations [41] (Methods). In the case of our actual device, the finite lengths of the taper sections lead to imperfect mode matching into the APCW near the band edge. As illustrated in Fig. 3a , the matching sections partially reflect an incident probe pulse and form a low finesse ( ) cavity around the APCW. These weak cavity resonances in the reflection spectrum near ν 2 are shown in Fig. 1c (without atoms) and complicate the spectra taken with atoms relative to the ideal case, as discussed below. In Fig. 3b,c , we measure distinctive reflection spectra with cold atoms under two configurations of the APCW. Figure 3b displays acquired near a resonance for the matching cavity where the reflectivity with no atom is very small (Methods). We observe an increased peak reflectivity . By comparison, with the matching cavity excited midway between two cavity resonances where the reflectivity with no atoms is , we observe decreased reflectivity with a minimum in Fig. 3b . These reflection spectra are in accord with those for a low finesse Fabry–Perot (FP) cavity containing a frequency-dependent intracavity absorber ( Fig. 3a ). In Fig. 3b with input frequency resonant with the FP cavity and no atoms, the transmission is high, and there is very small reflection (Methods). Atoms inside the PCW reduce light build-up by frequency-dependent atomic absorption, resulting in an increased reflectivity . By contrast, in Fig. 3c without atoms, the device reflectivity is larger due to the off-resonant drive of the FP and is reduced by intracavity atomic absorption, . The reflection spectra in Fig. 3b,c represent strong evidence for atomic interactions with the guided mode E 2 of the APCW. Although the cavity formed by the matching sections has a low finesse, R (Δ p ) nevertheless depends on the cavity detuning as predicted, that is, exhibiting approximately Lorentzian profiles for increased (decreased) for ν 2 a coincident with (midway between) the weak cavity resonances. Moreover, our numerical simulations as in Fig. 3d–f suggest that the blue-detuned E 1 mode performs three functions: excluding atoms from the exterior of the APCW, as in Fig. 3e ; guiding atoms into regions of large E 2 probe intensity near the centre of the unit cells, as in Fig. 3d, f ; and expelling atoms from the vicinity of other parts of the waveguide, for example, the single-nanobeam regions in Fig. 2b , leaving only the APCW region with significant atom–field interactions. Together, these considerations enable us to infer quantitatively the single-atom emission rate absent reflections from the tapered sections, as we now describe. Reflection measurements and theoretical fit To obtain quantitative information about atom–light coupling in the APCW region, we compare our measurements with a model based on transfer matrix calculations of the optical pathway to and from the APCW as illustrated in Fig. 3a . Details of the optical elements, including the coupling fibre, the supporting structures, and the APCW, are described in Methods and ref. 43 . Absent atoms, the optical characteristics of these various elements can be deduced from measurements of reflection spectra (for example, Fig. 1c and Methods). With atoms, free parameters are the average atom number within the APCW, the ratio for an atom at the centre of the probe mode E 2 , and the frequency shift δ 0 of the line centre ν 0 relative to free space, δ 0 = ν 0 − ν 2 a . Here atoms are drawn from a Poisson distribution and placed randomly along the APCW. Comparisons between measurements and our model for are given in Fig. 4 . For these data, the weak cavity formed by the matching sections has a small detuning Δ c ≃ 50 GHz from the midpoint between two resonances (free spectral range ~600 GHz). With atoms, the cavity detuning results in asymmetric, dispersive-like reflection spectra, which is captured by our model. From fits to the measured reflection spectra in Fig. 4 , we deduce that Γ 1D /Γ′ ≃ 0.35±0.1 and for loading from a free-space cloud of density ρ 0 . 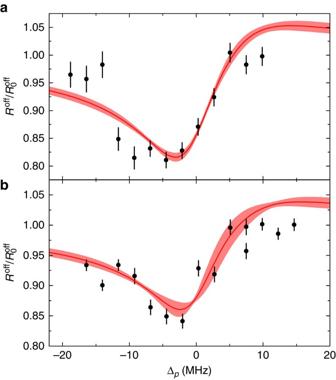Figure 4: Measured reflection spectra and theoretical fit for the APCW. Measured reflection spectra (circles) with free-space atomic cloud densitiesρ/ρ0=1 (a), and 0.75 (b) where the reflectivity with no atoms is. The full curves are fits with a model derived from transfer matrix calculations. Error bars for the data points reflect 1 s.d. estimated from the statistical uncertainties. We deduce that(a) and (0.36±0.1,0.76±0.13,0.48±0.07) (b). Here,ρ0=2 × 1010cm−3; Γ0/2π=5.2 MHz (decay rate in free space). The shaded band gives the uncertainty arising from the position of the matching cavity (Methods). Figure 4: Measured reflection spectra and theoretical fit for the APCW. Measured reflection spectra (circles) with free-space atomic cloud densities ρ / ρ 0 =1 ( a ), and 0.75 ( b ) where the reflectivity with no atoms is . The full curves are fits with a model derived from transfer matrix calculations. Error bars for the data points reflect 1 s.d. estimated from the statistical uncertainties. We deduce that ( a ) and (0.36±0.1,0.76±0.13,0.48±0.07) ( b ). Here, ρ 0 =2 × 10 10 cm −3 ; Γ 0 /2 π =5.2 MHz (decay rate in free space). The shaded band gives the uncertainty arising from the position of the matching cavity (Methods). Full size image The inferred value of Γ 1D allows us to determine for the atom–field interaction in our experiment, namely for an unpolarized atom. Together with the E 2 mode profile, the value of A m suggests that atoms are distributed in narrow regions around nm, which is consistent with our numerical simulations ( Fig. 3d–f ). The large ratio Γ 1D /Γ′ ≃ 0.35 implies a single-atom reflectivity | r 1 | ≃ 0.26, which is sufficient to give a nonlinear dependence of on the atom number observed in the measured spectra. We are thereby able to disambiguate the product into separate parameters in fitting our model to measurement. Saturation measurement To further investigate the nonlinear dependence of the reflection spectra on atom number, we measure reflection spectra for increasing values of probe power P in the E 2 mode for various values of . 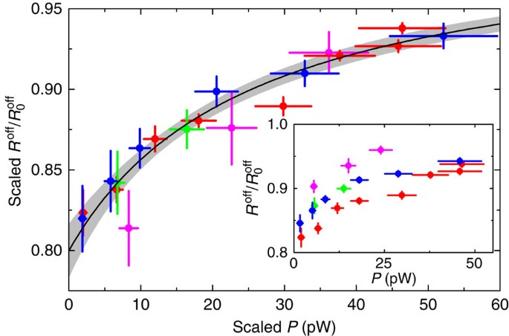Figure 5: Scaled reflection minimum as a function of averaged probe power inside the APCW. The saturation spectra (circles) are measured with four free-space densitiesρ/ρ0=1 (red), 0.81 (blue), 0.75 (green), 0.44 (magenta), and rescaled to a common free-space densityρ0≃2 × 1010cm−3; see text and Methods. The inset shows the saturation data without scaling. An empirical fit (solid curve) gives a saturation power of 22.7±2.2 pW. Error bars for the data points are 1 s.d. estimated from the statistical uncertainties and uncertainties of the fit to the model. The gray area shows 95% confidence band. Figure 5 presents results for from a series of measurements as in Fig. 4 for increasing P with the plotted points corresponding to the minima of versus Δ p for each spectrum. The inset of Fig. 5 displays four sets of measurements showing that saturation of the atomic response (that is, with increasing P ) requires higher power as the density is increased (that is, increasing ). Figure 5: Scaled reflection minimum as a function of averaged probe power inside the APCW. The saturation spectra (circles) are measured with four free-space densities ρ / ρ 0 =1 (red), 0.81 (blue), 0.75 (green), 0.44 (magenta), and rescaled to a common free-space density ρ 0 ≃ 2 × 10 10 cm −3 ; see text and Methods. The inset shows the saturation data without scaling. An empirical fit (solid curve) gives a saturation power of 22.7±2.2 pW. Error bars for the data points are 1 s.d. estimated from the statistical uncertainties and uncertainties of the fit to the model. The gray area shows 95% confidence band. Full size image The observed saturation behaviour can be scaled into a common curve using the dependence of cooperative atomic emission on atom number . We assume that R off ( P )= R off ( P / P sat ) and that the saturation power P sat depends on the average total decay rate as with Γ 1D /Γ′=0.35±0.1, as determined from our measurements in Fig. 4 with P →0. We rescale the probe power (horizontal axis) for each density in the inset of Fig. 5 to a common density ρ 0 . Likewise, (vertical axis) is rescaled using the density dependence derived from our transfer matrix model (Methods), with . The approximate convergence of the data to a common curve in Fig. 5 supports our rudimentary understanding of the underlying atom–field interactions in the APCW, including that the observed line shapes for the data in Fig. 5 taken at higher power (not shown) are predominately homogeneously broadened. To estimate the saturation power in the APCW, we adopt an empirical form for the saturation behaviour . From the fit in Fig. 5 , we determine pW and as shown in Fig. 4(a) . Combining with the measured effective mode area, we find the saturation intensity I sat = P sat / A m ≃ 5.2 mW cm −2 , close to the expected value , where I s0 =2.7 mW cm −2 is the free-space saturation intensity. We have realized a novel APCW device for interfacing atoms and photons. The measured coupling rate Γ 1D (quoted absent Purcell enhancement and inhibition due to an external cavity) is unprecedented in all current atom–photon interfaces, whether for atoms trapped near a nanofiber [27] , [28] , [29] , one atom in free space [45] , or a single molecule on a surface [46] . For example, in ref. 26 a drop in transmission ≃ 0.02 is observed for single atoms trapped outside a photonic crystal cavity. In our work without trapping, we observe a dip in reflection ≃ 0.25 for since atoms are channelled to near the peak of the probe mode in the centre of unit cells with stronger interactions. Further improvements to the APCW include active tuning of the band edge to near an atomic resonance to achieve an increase ≳ 50-fold in Γ 1D [41] , [47] , although we are mindful of challenges presented by disorder-induced localization [48] , [49] . Other opportunities could be tuning to place the atomic resonance within the band gap to induce long-range atom–atom interactions [4] , [16] , [17] , [18] . By optimizing the power and detuning of the E 1 trap mode, we should be able to achieve stable atomic trapping and ground state cooling [41] , [50] , [51] . By applying continuous on-site cooling to N ≫ 1 atoms, we expect to create a 1D atomic lattice with single atoms trapped in unit cells along the APCW, thus opening new opportunities for studying novel quantum transport and many-body phenomena [5] , [6] , [7] , [8] , [9] , [10] , [11] , [12] , [13] , [14] , [15] , [16] , [17] , [18] . Design principle An APCW is designed on a chip in order to observe strong atom–light interactions, as illustrated in Supplementary Fig. 1 . The APCW interacts with a cloud of caesium atoms trapped in a magneto-optical trap (MOT) that is centred on the photonic crystal. The APCW (see inset V of Supplementary Fig. 1 ) consists of two parallel nanobeams with sinusoidal corrugations on the outer edges [43] . The atoms are guided into the centre of the two nanobeams by a scheme that takes advantage of the TE-like modes ( y -polarized) near the band edges [52] . Their highly symmetric mode profiles near the dielectric and air bands at frequencies ( ν D , ν A ) and the proximity to the resonant frequencies ( ν 1 , ν 2 ) of the caesium D 1 , D 2 lines allow us to create strong dipole potentials with small optical power (<10 μW) in the E 1 mode, while achieving large atom–photon coupling in the E 2 mode. See Fig. 1d,e for calculated mode profiles. The corrugations in the APCW are used rather than the more traditional holes because the corrugation amplitude can be patterned more accurately than hole radii, resulting in more accurate alignment of the band gaps and better adiabatic tapers. The outside-corrugated double-beam design used in this work allows superior band edge positioning by placing the modulation of the dielectric away from the strong-field region in the centre of the waveguide, hence reducing the sensitivity of band edge frequencies to the modulation geometry parameter imprecision. This design also avoids enclosed hole-based geometry, which is difficult to fabricate using available lithography and etching techniques. The design also enables us to build vanishingly small amplitude modulations required for the gradual tapers. The waveguide is made from 200-nm thick stoichiometric SiN with index n =2.0 (ref. 43 ). SiN is a widely used material in standard silicon-based fabrication processes, which we have chosen for its low absorption for the Cs D-line transition wavelengths where Si itself is opaque. Its high intrinsic stress and Young's modulus makes it mechanically robust, hence it was chosen instead of the also low-loss SiO 2 . The degrees of freedom for the APCW are the gap g , lattice constant a , width w (inner-edge to centre of peaks), and tooth amplitude A . The APCW has 260 cells, gap 250 nm, width 173 nm and tooth amplitude 132 nm. The photonic crystal is tapered on both sides into an unpatterned (translationally invariant) double nanobeam. The length and profile of the tapering determines the reflections from the edges of the APCW. The taper used here has 40 cells, and is carefully designed such that the band gap symmetrically opens about 873 nm, which is between the caesium D 1 and D 2 lines. The profile and the unpatterned double waveguide width are chosen to minimize reflections from the APCW edge. In order to provide optical access for the trapping and cooling laser beams, the SiN waveguides are suspended across a 1 mm long, 3 mm wide through window on the chip, shown in Fig. 2a , and the APCW (see Supplementary Fig. 1 ) is positioned at the centre. The suspended waveguide extends beyond the window into a V-groove etched into the Si substrate and then reduces in width for efficient coupling to a conventional optical fibre [44] (sections I–II of Supplementary Figs 1 and 2 ). The silicon anisotropic etch that forms the window also forms the V-groove, which serves to centre the fibre to the waveguide. The far end of the waveguide is extended to a fan shape and terminated into the substrate to minimize reflection (section VI). Atom–photon coupling To characterize the strength of atom–photon coupling, we calculate the effective mode area for an atom at where a is a lattice constant of 371 nm and the integration runs over the space occupied by a unit cell. Supplementary Fig. 3 shows plotted at the central x =0 plane. For single atoms channelled to the centre of unit cells, we have A m ( 0 )=0.24 μm 2 . To estimate the atomic emission rate into the guided mode, we use , where Γ 0 is the atomic decay rate in free space, σ the radiative cross-section, and n g the group index at ν 2 . When the band edge frequency ν A is placed near ν 2 , we expect n g >>1 due to the slow light effect [41] ; for the current device where c the speed of light, Δ ν the distance between neighboring resonant dips and L Phc the length of APCW (see Supplementary Fig. 1b ). Note that due to our small band edge (Δ ω / ω 0 ~0.04), we would have to operate much closer to the band gap than in our current experiment in order to observe a significant slow light effect (for example, n g >10). For atoms guided to the centre of unit cells and driven by the F =4, m F =0↔ F ′=5, m F ′ =0 transition, σ ≃ 5/9 × 3 λ 2 /2 π , where λ =852 nm is the free-space wavelength of the Cs D 2 line, with then Γ 1D /Γ 0 ≃ 0.4 n g ; for unpolarized atoms, we calculate an averaged Γ 1D /Γ 0 ≃ 0.29 n g . Device characterization Supplementary Fig. 4a shows a schematic of the setup for device characterization. The reflection spectrum near the band gap is measured by sending a broadband light source into the device via the coupled optical fibre, and then recording the reflection signal with an optical spectrum analyser. The signal is then normalized by the power spectral density of the light source after considering the loss of each optical element. Finer reflection spectra around the D 1 and D 2 lines are measured by scanning the frequency of narrow bandwidth diode lasers. The polarization in the device is aligned to the TE-like mode by observing the polarization-dependent scattering from the first tether in the coupler, or equivalently by maximizing the reflected signal, since the transverse magnetic mode band gap is located at a higher frequency. Supplementary Fig. 4b shows the measured reflection spectra around the band gap. The gray curve shows the original data that has a fast fringe (free spectral range ~50 GHz) resulting from the (parasitic) etalon formed from the cleaved fibre end-face and the first matching taper. The red curve shows the smoothed reflection spectrum that approximately represents the response of the APCW without the influence of the reflection from the fibre end-face. Device model Due to imperfection of the adiabatic tapering, the terminal regions of the APCW form a low finesse cavity. When atoms couple to light in the APCW, the reflected spectrum depends on the position of the frequency ν 2 on the cavity fringe and can take on dispersive line shapes. Further complicating the picture is the presence of a fast ~50 GHz fringe due to the parasitic etalons formed by the fibre end-face, tethers, and the APCW band edges near ν D , ν A . In order to fit the reflected atomic signals, a full model that incorporates all of these elements is developed using the transfer matrix method [52] , [53] as shown in Supplementary Fig. 5 . A transfer matrix represents each element, and the reflection, transmission and loss coefficients are determined by both experiment and FDTD simulations [54] . The light is coupled into the device by matching the modes of a 780HP single mode fibre (mode field diameter 5 μm) to a 130 nm wide rectangular SiN waveguide (parts I–II in Supplementary Figs 1b and 2 ). The fibre end-face reflects 3.8% power due to the index mismatch. A 90 nm wide tether anchors the coupling waveguide 5 μm from the free (input) end of the waveguide, which has a theoretical transmission of 87% and reflection 0.8%. The waveguide width tapers to 200 nm over 300 μm in order to better confine the light to the dielectric, and then the light propagates through the region of the support rails (part III in Supplementary Fig. 1b ) to the APCW at the centre of the window. Our numerical simulations show that the taper, support rails and guide should have negligible loss and reflection. The loss in these sections is measured to be 22% per mm for a similar device. The details of loss mechanism are currently under investigation. The total loss from the fibre face to the waveguide can be estimated experimentally by measuring the reflected signal for frequencies within the band gap, assuming the reflectivity of the APCW from numerical simulations is ~99%. By fitting our model to the envelope of the reflection spectrum inside the band gap, we obtain the overall transmission efficiency from the internal face of the fibre to the input of the APCW to be T t ≃ 0.60, including propagation losses in the nanobeam. The tapers of the APCW (represented by the matching mirrors in Supplementary Fig. 5 ) also reflect near the band edge. There is also loss inside the APCW due to fabrication disorder and absorption. Near the Cs D 2 line, as shown in the Supplementary Fig. 4c , the fitted spectrum (solid gray line) yields the reflection and transmission of the matching sections of the APCW, ( R pc =0.28, T pc =0.72), the slope of the reflection of the APCW d R pc /d λ =0.082 nm −1 , and the one-way transmission inside the APCW, T APCW =0.40±0.02. At the bottom of the fast fringe, for the experiment presented in Fig. 3b , measured reflection without atoms is and reflection in front of M 1 estimated from the device model is ; in Fig. 3c , and estimated reflection in front of M 1 , . The role of disorder in the APCW The presence of fabrication imperfection and disorder do not significantly alter our analysis, which we discuss in the following section. It is well known that disorder in PCWs can dramatically modify the optical properties by creating localized modes with high quality factors, resulting in large Purcell enhancement for an emitter within a localization volume [48] , [49] . In Figure 1c , we observe variations in the positions and sizes of the cavity resonances near the band edges compared with the ideal case that are likely due to disorder from imperfect device fabrication. However, for our analysis to determine Γ 1D and , the only assumption required is that the fields internal to the APCW near the caesium D 2 line behave as spatially extended modes over the entire length of the APCW. In this section, we present evidence that this is indeed the case, with effects due to disorder-induced localization playing a minor role. Many groups have observed non-dispersive regimes in which the localization length L D for light becomes smaller than the length L PCW of the PCW. The non-dispersive regime onsets for relatively large group indices n g ≥20 (refs 55 , 56 ). By contrast, our device is operated in a regime where n g ≈2, much lower than where localization has been observed. In addition to having a low group index, we have determined from SEM images that the disorder on the sidewalls of our SiN devices has s.d. σ ≈2 nm, which is consistent with state-of-the-art fabrication techniques. For our measured low group index and small disorder, multiple analyses in the literature suggest that we are far from the non-dispersive regime. By performing full 3D FDTD simulations [54] of the APCW with and without disorder, we have confirmed that the measured disorder in our devices does not result in localized modes. The disorder is introduced as Gaussian fluctuations of s.d. σ =2 nm for sidewall fluctuations (with a correlation length of 100 nm), as determined from SEM images. Similar to our measured devices, we observe variations in the positions and linewidths of the cavity resonances formed by the taper sections near the band edges and mode profiles extend over the entire length of the APCW, which is consistent with the ideal case. Even for the cavity resonance closest to the band gap, where the group index is n g ~10, we observe no signatures in the intracavity intensity that would suggest localization on a scale shorter than the APCW length. We have also observed evidence that cavity resonances for reflected light correspond to intracavity modes that extend over the entire length of the APCW by imaging spatially resolved scattered light along the APCW. For devices similar to the one used in our work, we have observed intensity profiles consistent with the cavity resonances and antiresonances near the band edges. For example, at the third cavity resonance from the band gap, we observe three bright antinodes along the photonic crystal. As show in ref. 43 , by measuring the scattered light at various positions along the APCW, we can distinguish between even and odd cavity resonances. Furthermore, if there were to be a localized mode L D < L PCW that has otherwise escaped our detection (for example, with L D ≪ L PCW and a concomitant non-negligible Purcell effect), such a mode would lead to reflection spectra that are incompatible with our observations. Roughly speaking, for fixed atomic density around the APCW (which we know from shot-to-shot measurements by absorption imaging of the cold atom cloud), a mode of length L D would interact with an atom number f times smaller than is the case for interactions over the entire length L PCW , where f = L D / L PCW <1. Hence to create comparable absorption leading to the observed reflection dip, the atomic coupling strength Γ Purcell would need to be increased beyond Γ 1D for the entire APCW by roughly 1/ f >1 for atomic interaction with the localized mode (assuming Purcell enhancement for the localized mode comparable with that for the APCW with a finesse ). Such an increase in coupling by roughly 1/ f (from Γ 1D to Γ Purcell ) and decrease in average number by ~ f (from to ) would be incompatible with our observations and modeling. For example, the linewidth for the observed reflection spectrum would be increased by ~1/ f >>1 for L D ≪ L PCW , which is inconsistent with our measurements. In summary, the three pieces of evidence given above strongly suggest that cavity resonances in our reflection spectrum are not associated with localized modes of spatial extent smaller than our photonic crystal. It is of course possible that other forms of disorder are playing a role in the photonic crystal. An example is disorder from long-range fluctuations in the device dimensions that could smooth the observed band edges but that would not induce a localized mode (as we have confirmed by numerical simulation). The consequences of other forms of disorder are currently under investigation. The main point to stress is that our analysis requires only that the observed structure in reflection spectra near the caesium D 2 line is associated with cavity resonances for which the intracavity intensity extends over the length of the PCW. Simulations of relative density To estimate a relative atomic density near the APCW with a guiding potential, we calculate a relative density , where ρ 0 is a free-space cloud density, with a Monte Carlo simulation of 5 × 10 6 trajectories of thermal atoms with a temperature of 20 μK (ref. 57 ). For the simulations, the Casimir–Polder potential for the APCW is computed numerically following ref. 41 , with an example cut shown in Supplementary Fig. 6a . The dipole potential of the blue-detuned guided mode near ν 1 is calculated by using the mode function obtained with MIT Photonic Band package [58] . Trajectories are obtained by numerically solving the equation of motion with force of . The relative density is inferred from atomic flux crossing each grid. Note that velocity-dependent forces of polarization-gradient cooling are not included in the simulations. In Fig. 1f and Supplementary Fig. 6b , we use a guided mode at the band edge k D , x = π / a at ν D with total power of 1 μW and 10 GHz blue-detuning from F =4↔ F ′=4 transition frequency of D 1 line, which has zero intensity at the centre of unit cells of the APCW. Thus, atoms are channelled into unit cells by the combination of Casimir–Polder and optical dipole force. The relative density at the centre of unit cells is . In Fig. 3d–f and Supplementary Fig. 6c , we use experimentally excited with k 1, x near ν 1 (Cs D 1 line), which is ~1% below the band edge k D , x . Due to the small deviation from the band edge, the intensity of the mode field near ν 1 has a small bump at the centre of the unit cells, which for blue detuning prevents atoms from being channelled to the centre. In addition, the intensity of has a longitudinal component E x along the propagation direction, which is π /2 out-of-phase with the transverse components. As a consequence, the polarization of is elliptical everywhere except for the central y =0 plane of unit cells due to TE symmetry. The resulting guiding potential has vector shifts due to the ellipticity of , which lead to m F -dependent guiding potentials. Since the centre of guiding channel for | m F | ≠0 states moves from y =0 to | y | >0 due to a stronger fictitious magnetic field (along z ) closer to the structure, the guiding efficiency from optical dipole forces is reduced as | m F | increases. Figure 3d–f displays , where is simulated relative atomic density with a guided potential for m F =0, and Γ 1D ( 0 ) is a decay rate into the APCW at the centre of unit cells. Due to the small deviation from the band edge and the resulting potential ‘bump’, atoms are localized around >100 nm from the centre of unit cells. We note that, in the case of Supplementary Fig. 6c , adding to U dipole the dipole potential from a weak red-detuned mode can help overcome the potential bump in the gap centre and can create a stable trapping condition. This scheme is currently under investigation and will be presented elsewhere. Experimental procedure To prevent caesium contamination of the APCW due to the background vapor pressure, our vacuum system consists of a source chamber and a science chamber, connected via a differential pumping stage. The source chamber runs in a standard MOT loaded from the background Cs vapor. From the source MOT, a pulsed push beam extracts a flux of cold atoms that is slow enough to be recaptured in a science MOT located in the UHV region [59] . We load a science MOT for 1 s and compress it for a duration of 50 ms (ref. 60 ). We then obtain a cloud of cold atoms with a peak density of ~1 × 10 11 cm −3 and a temperature of 40 μK about 1 cm away from the APCW of a silicon chip. In order to transport cold atoms near the APCW, we cool atoms in the moving frame towards the APCW by abruptly changing the centre of magnetic quadrupole field [61] . After shutting off cooling beams, a cloud of atoms freely propagates towards the APCW. By turning on additional MOT beams at the time atoms fly near the APCW, we cool and recapture propagating atoms with an efficiency of ~40%. After applying polarization-gradient cooling, we obtain a cloud of cold atoms with a peak number density of ρ 0 ~2 × 10 10 cm −3 , spatially overlapped with the APCW. An overview of reflection measurements in our experiment with cold atoms near the APCW is given in Supplementary Fig. 7 . A blue-detuned guiding beam with power ~0.6 μW and detuning of +10 GHz from D 1 ( F =4↔ F ′=4) at k 1, x =0.99 k D , x is sent into the device, which is kept on throughout the experiment. The probe pulse is combined with the guiding beam by a volume Bragg grating and then couples to the APCW via a fibre beam splitter with T =99% and R =1%. The reflected probe signal from the APCW is efficiently picked up by the fibre beam splitter through the transmission path. An additional volume Bragg grating at the output reflects the return probe beam, which allows us to measure the probe pulses with the guiding beam on. A pair of λ /2 and λ /4 waveplates in each path is used for aligning the polarization to only excite the TE-like mode. To maximize the signal-to-noise ratio, we perform reflection measurements with atoms after aligning the bottom of the fast fringe to the Cs D 2 line, where the probe field is maximized inside the parasitic cavity formed by the fibre end-face and the APCW region; see Supplementary Fig. 8a . The alignment of the fast fringe can be tuned by sending an additional few μW of heating beam to heat up the device and adjust the optical path length between the fibre end-face and the APCW region. The heating beam runs at frequency ν > ν D inside the band gap and is ≃ 5 nm detuned from D 1 line, thus does not interfere with atom–light interaction in the APCW region. Model of reflection spectrum of atoms Reflection spectra of guided atoms are obtained by including transfer matrices for atoms [62] in the device model. Guided atoms inside the APCW are drawn from a Poisson distribution with mean atom number and randomly placed at the centre of unit cells along the APCW. Each of the two matching sections that terminate the APCW partially reflects light near the band edge, as depicted in Supplementary Fig. 5 . Together the matching sections form a cavity around the APCW (denoted by M 1 , M 2 in Supplementary Fig. 5 ), whose cavity length has a frequency dependence. We incorporate the uncertainty of the location of the matching mirrors and resulting cavity relative to the APCW into our model. This uncertainty gives rise to a variation in the reflection spectra from our model, which is given by the thickness of the lines shown in Supplementary Fig. 8 . The wave vector of probe frequency k p , x is ≃ 2% from the band edge at k A , x = π / a as shown in Fig. 1b . In the case of more than one atom coupled to the APCW, the mismatch between k A , x and k p , x causes dephasing since the accumulated phase between atoms is not an integer multiple of π . Due to the moderate one-way transmission of T APCW ≃ 0.40 inside the APCW as described in Section III, the cooperative effect of two atoms is sensitive to how loss occurs inside of the APCW. Here, we consider two limiting cases: (i) uniform absorption along the APCW, and (ii) loss at the first matching mirror. In the case of (i), due to uniform loss along the APCW, only nearby atoms interact equally with the probe field. Thus, cooperative effects survive despite of the mismatch of k p , x and k A , x . On the other hand, in the case of (ii), all atoms contribute equally and cooperative effects are washed out due to the phase mismatch for propagation with k p , x as compared with k A , x for the unit cell. Given our current limited knowledge of the microscopic details of the loss mechanisms within the APCW, the models (i, ii) provide a means to estimate the uncertainties in our inferences of Γ 1D /Γ′ and average atomic number based upon comparisons of our data with the models. For the cases shown in Supplementary Fig. 8 , the model fits lead to the following: (i) Γ 1D /Γ′=0.31±0.05 and average atom number in (b), and (ii) Γ 1D /Γ′=0.41±0.04 and in (c). From four sets of data as in Supplementary Fig. 8 , taken for comparable atomic densities, we make fits based upon the two models (i) and (ii). We average results for parameters determined from the fits to arrive at the values quoted, namely Γ 1D /Γ′=0.32±0.08, and δ 0 /Γ 0 =0.13±0.27. How to cite this article: Goban, A. et al. Atom–light interactions in photonic crystals. Nat. Commun. 5:3808 doi: 10.1038/ncomms4808 (2014).